Iron-catalyzed carboazidation of alkenes and alkynes Carboazidation of alkenes and alkynes holds the promise to construct valuable molecules directly from chemical feedstock therefore is significantly important. Although a few examples have been developed, there are still some unsolved problems and lack of universal methods for carboazidation of both alkenes and alkynes. Here we describe an iron-catalyzed rapid carboazidation of alkenes and alkynes, enabled by the oxidative radical relay precursor t -butyl perbenzoate. This strategy enjoys success with a broad scope of alkenes under mild conditions, and it can also work with aryl alkynes which are challenging substrates for carboazidation. A large number of diverse structures, including many kinds of amino acid precursors, fluoroalkylated vinyl azides, other specific organoazides, and 2 H -azirines can be easily produced. Amino acids, the basic building blocks of proteins are being used increasingly in bio-relevant modification of proteins and pharmaceutical applications. Development of more versatile methods to provide useful but synthetically challenging amino acid frameworks from chemical feedstocks is always highly desired [1] , [2] , [3] , [4] . Carboazidation of alkenes and alkynes holds the promise to construct valuable molecules including amino acid precursors and has therefore attracted much attention recently. Although several carboazidations of alkenes have been developed by Huang [5] , Renaud [6] , [7] , Liu [8] , Masson [9] , Zhu [10] , Jiao [11] and Xu [12] , there are some unsolved problems in this field. How to realize the carboazidation reaction using nontoxic, inexpensive and readily available reagents with a broad scope of olefins remains a question. In addition, the carboazidation of alkynes is even more challenging than carboazidation of alkenes (Fig. 1 a). There is only one successful carboazidation of alkynes reported by Liu [13] which works for single carbon functionality, i.e., a trifluoromethyl group using Togni’s reagent (Fig. 1 b). The reason for the lack of methods for carboazidation of alkynes might be attributed to the relative lower efficiency of incorporation of azido species compared to other competing reactions. The development of carboazidation of alkenes and alkynes is significantly important from the synthetic point of view. Fig. 1 Carboazidation of alkenes and alkynes. a Previous arts on carboazidation of alkenes. b Previous arts on carboazidation of alkynes. c This work: carboazidation of alkenes and alkynes Full size image t -Butyl perbenzoate (TBPB) is a commercially available and inexpensive oxidant frequently used as a precursor of the t -butoxyl radical [14] , [15] , [16] , [17] , [18] , [19] , [20] , [21] , [22] . Lately, TBPB has been proved to be a good source of methyl radical by Yu [23] and our group [4] , [24] , [25] . Although our understanding of the selective formation of methyl radicals is limited, we found previously that in the presence of Fe(OTf) 2 or Fe(OTf) 3 , the methyl radical is formed exclusively. We envisioned that TBPB could serve as a polyfunctional reagent for the carboazidation of alkenes and alkynes. Herein, we report our development of a versatile iron-catalyzed rapid carboazidation of both alkenes and alkynes, enabled by TBPB (Fig. 1c ). Carboazidation of alkenes We investigated the reaction parameters for carboazidation in the presence of TBPB and found that ferrous trifluoromethanesulfonate (Fe(OTf) 2 , ferrous triflate) is optimal (Fig. 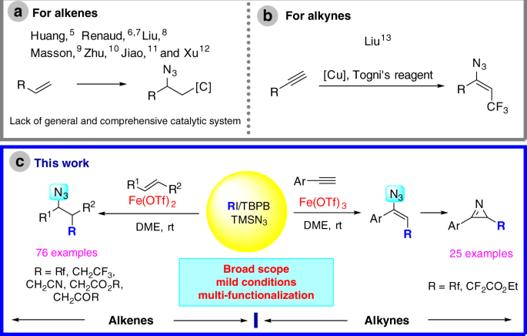Fig. 1 Carboazidation of alkenes and alkynes.aPrevious arts on carboazidation of alkenes.bPrevious arts on carboazidation of alkynes.cThis work: carboazidation of alkenes and alkynes 2 , see details in Supplementary Table 1 and Supplementary Figures 2 – 4 ), delivering the corresponding product 3 in 89% yield at rt with DME (dimethoxyethane) as the solvent and azidotrimethylsilane (TMSN 3 ) as the azidation reagent. Possible by-products 4 , 4 ′, and 4 ″ were not observed. Fig. 2 Optimized conditions for carboazidation of alkenes. Fe(OTf) 2 (5 mol%), 1a (0.5 mmol), 2a (1.0 mmol), TMSN 3 (1.0 mmol), TBPB (1.0 mmol) in DME (2 mL) at rt for 3 min under an N 2 atmosphere Full size image With the optimized conditions in hand, we studied the scope of the reaction with alkyl iodides (Fig. 3 and Supplementary Figures 5 – 34 ). Fluoroalkyl iodides were examined first and the corresponding fluoroalkyl-azidation products ( 5 – 10 ) were obtained in high yields [26] . The reaction of styrene with iodoacetonitrile proceeds smoothly, affording the corresponding product ( 11 ) in 86% yield. Reactions with ethyl iodoacetates affords products ( 12–14) with the yield ranging from 71–85%. With 1-iodo-3,3-dimethylbutan-2-one the reaction delivers the azide ( 15 ) in 61% yield. Three electron rich alkyl iodides, i.e., 1-chloro-4-iodobutane, 1-iododecane and 2-iodobutane are not effective in this reaction as the direct azidation of alkyl iodides to form alkyl azides occurs. It should be noted that the reactions with perfluoroalkyl iodides are very fast, completing in 10 min in many cases. Fig. 3 Scope of alkyl iodides. General reaction conditions: Fe(OTf) 2 (3–5 mol%), 1a or 1b (0.5 mmol), 2 (0.65–1.0 mmol), TMSN 3 (0.7–1.0 mmol), TBPB (0.75–1.0 mmol) in DME (2 mL) at rt under an N 2 atmosphere. a Instead of TBPB, lauroyl peroxides (LPO, 0.75 mmol) was applied. b 50 °C Full size image Subsequently, we studied the substrate scope of olefins (Fig. 4 and Supplementary Figs. 35 – 189 ). As examples, α -azido esters ( 16–27 in Fig. 4a ), β- azido esters ( 28–37 in Fig. 4b ), γ- azido esters ( 38–63 in Fig. 4c ), other azido acid derivatives ( 64–69 in Fig. 4d–g ) and organoazides ( 70–75 in Fig. 4h ) were obtained. The functional group compatibility of this reaction is good: a series of functional groups, such as halogen, ester, carboxylic acid ( 69 ), and free hydroxyl group ( 74 ) are tolerated under the reaction conditions. Both terminal and internal alkenes ( 28–37, 58 , and 65 ) are compatible with the reaction. The carboazidation reactions of 1-octene with iodomethane and iodobutane are not successful under the reaction conditions. Fig. 4 Scope of alkenes. a Synthesis of α-azido esters. b Synthesis of β-azido esters. c Synthesis of γ-azido esters. d Synthesis of α,γ-azido esters. e Synthesis of an α,β-azido ester. f Synthesis of an α,β,γ-azido ester. g Synthesis of an azido acid. h Synthesis of other organoazides. General reaction conditions: Fe(OTf) 2 (5 mol%), 1 (0.5 mmol), 2 (0.65–1.0 mmol), TMSN 3 (1.0 mmol), TBPB (1.0 mmol) in DME (2 mL) at rt under an N 2 atmosphere. Isolated yields. dr values were determined by 1 H NMR Full size image To highlight the synthetic applications, 8 , 19 and 78 were reduced to amine 76 [11] , amino acid 77 [26] and pyrrolidinone 79 , respectively (Fig. 5 and Supplementary Figs. 190 – 199 ). Fig. 5 Applications of carboazidation products. a Reduction to amine. b Reduction to α-amino acid. c Cyclization to pyrrolidinones Full size image Carboazidation of alkynes Vinyl azides (1-azidoalkenes) [27] , [28] are versatile building blocks in organic synthesis and have been used in many transformations to synthesize bioactive alkaloids and heterocycles [29] , [30] , [31] , [32] , [33] , [34] , [35] , [36] . Although the carboazidation of alkynes can difunctionalize alkynes, affording 1-azidoalkenes which can be subsequently converted to 2 H -azirines, reports of such efficient methods are rare [13] , and accordingly, we studied the carboazidation of alkynes. After carefully screening the reaction conditions, Fe(OTf) 3 was found to be the best catalyst, producing a carboazidation product ( 81 ) while avoiding the formation of the atom-transfer radical addition (ATRA) product ( 81 ′) (Fig. 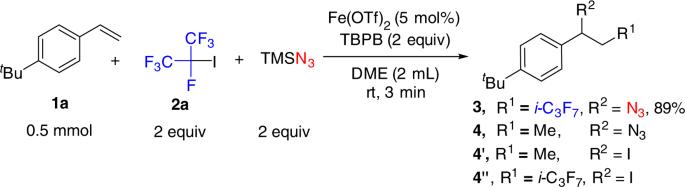Fig. 2 Optimized conditions for carboazidation of alkenes. Fe(OTf)2(5 mol%),1a(0.5 mmol),2a(1.0 mmol), TMSN3(1.0 mmol), TBPB (1.0 mmol) in DME (2 mL) at rt for 3 min under an N2atmosphere 6a , see details in Supplementary Table 2 and Supplementary Figs. 200 – 208 ). In view of the broad synthetic utilities of 2 H -azirines, the conversion of vinyl azides to 2 H -azirines was studied. It was found that compound 81 could be converted into a 2 H -azirine ( 82 ) in toluene at 120 °C (Fig. 6b ). Fig. 6 Carboazidation of alkynes. a Optimized reaction conditions. b Cascade transformation of vinyl azide to 2 H -azirine Full size image With these conditions identified, we studied the substrate scope regarding alkyl iodides and alkynes. The results are shown in Fig. 7 and Supplementary Figs. 209 – 283 . Fluoroalkyl iodides and aryl alkynes react well in these transformations. Reaction of 1-iododecane with ethynylbenzene does not deliver the desired product. As an example, reaction of 1-octyne delivers only the ATRA product (107 ) [37] in 42% yield. Fig. 7 Substrate scope of carboazidation of alkynes and further transformation to 2 H -azirines. General reaction conditions: Fe(OTf) 3 (0.025 mmol), alkyne (0.5 mmol), RI (0.75 mmol), TMSN 3 (1.0 mmol), TBPB (1.0 mmol) in DME (2 mL) at rt for 5–20 min and then in toluene at 120 °C for 10 min under an N 2 atmosphere. Isolated yields Full size image To highlight the synthetic applications of this method further, vinyl azides and 2 H -azirine were converted to 108 [38] 109 [39] and 110 [40] in high yields (Fig. 8 and Supplementary Figs. 284 – 295 ). 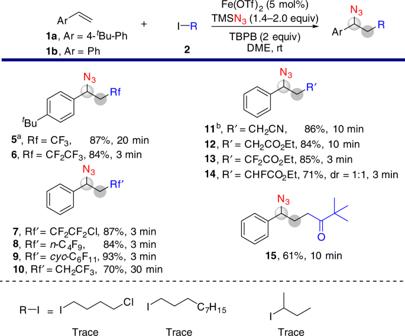Fig. 3 Scope of alkyl iodides. General reaction conditions: Fe(OTf)2(3–5 mol%),1aor1b(0.5 mmol),2(0.65–1.0 mmol), TMSN3(0.7–1.0 mmol), TBPB (0.75–1.0 mmol) in DME (2 mL) at rt under an N2atmosphere.aInstead of TBPB, lauroyl peroxides (LPO, 0.75 mmol) was applied.b50 °C The geometry of vinyl azides was confirmed by X-ray crystallographic analysis of product 109 (see details in Supplementary Figure 1 and Supplementary Table 3 ). Fig. 8 Further synthetic transformations. a Synthesis of 1,2,3-triazoles. b Synthesis of aziridine Full size image In summary, we have developed a carboazidation of alkenes and alkynes enabled by TBPB. This key transformation has been successfully used to afford various valuable structural skeletons, including many amino acid precursors, vinyl azides and 2 H -azirines. It is noteworthy that this carboazidation works for both alkenes and alkynes with multiple carbon functionalities. Typical procedure for carboazidation of alkenes Fe(OTf) 2 (9 mg, 0.025 mmol) was added to a dried Schlenk tube equipped with a magnetic bar. This tube was then flushed with N 2 gas (3 times) and an N 2 atmosphere was maintained using an N 2 balloon. 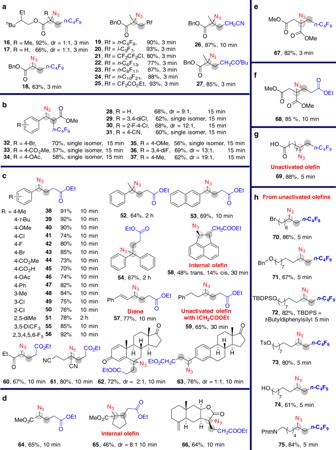Fig. 4 Scope of alkenes.aSynthesis of α-azido esters.bSynthesis of β-azido esters.cSynthesis of γ-azido esters.dSynthesis of α,γ-azido esters.eSynthesis of an α,β-azido ester.fSynthesis of an α,β,γ-azido ester.gSynthesis of an azido acid.hSynthesis of other organoazides. General reaction conditions: Fe(OTf)2(5 mol%),1(0.5 mmol),2(0.65–1.0 mmol), TMSN3(1.0 mmol), TBPB (1.0 mmol) in DME (2 mL) at rt under an N2atmosphere. Isolated yields. dr values were determined by1H NMR A thoroughly mixed solution of alkene (0.5 mmol), alkyl iodide (0.65–1.5 mmol), TMSN 3 (0.7–1.7 mmol) and TBPB (0.75–1.75 mmol) in DME (2 mL) was added to the catalyst by syringe and the mixture was stirred vigorously for 3–120 min at the appropriate temperature. After completion of the reaction, judged by TLC, the solvent was evaporated and the residue was purified by flash chromatography on silica gel using petroleum ether and EtOAc to give the corresponding product. Typical procedure for carboazidation of alkynes Fe(OTf) 3 (12.7 mg, 0.025 mmol) was added to a dried Schlenk tube equipped with a magnetic bar. Then this tube was flushed with N 2 (3 times) and an N 2 atmosphere was maintained using an N 2 balloon. 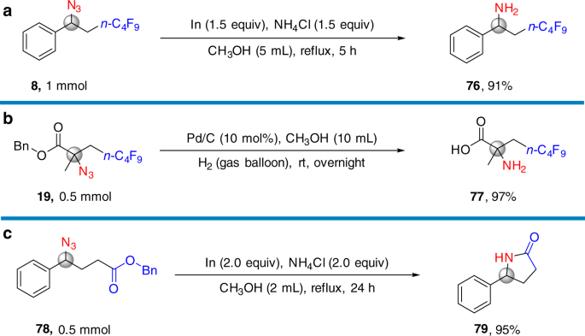Fig. 5 Applications of carboazidation products.aReduction to amine.bReduction to α-amino acid.cCyclization to pyrrolidinones A thoroughly mixed solution of alkyne (0.5 mmol), R f I (0.75 mmol), TMSN 3 (1.0 mmol) and TBPB (1.0 mmol) in DME (2 mL) was added to the catalyst by syringe and the mixture was stirred vigorously for 5–20 min at rt. After completion of the reaction, judged by TLC, the volatile compounds were removed by pump and the residue was dissolved in toluene (3 mL). 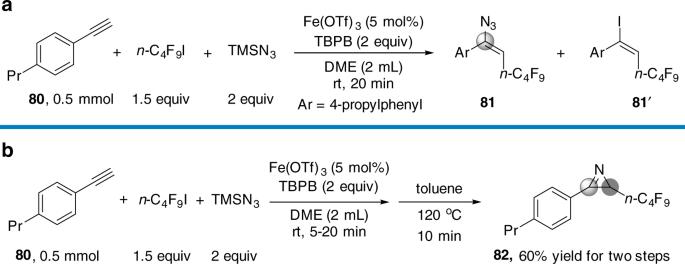Fig. 6 Carboazidation of alkynes.aOptimized reaction conditions.bCascade transformation of vinyl azide to 2H-azirine The resulting mixture was then stirred at 120 °C for 10 min. 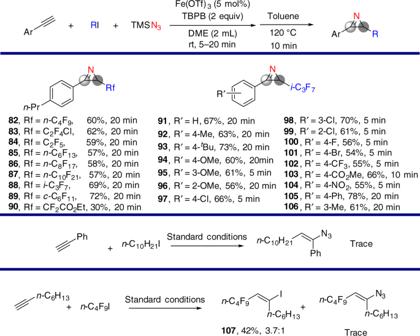Fig. 7 Substrate scope of carboazidation of alkynes and further transformation to 2H-azirines. General reaction conditions: Fe(OTf)3(0.025 mmol), alkyne (0.5 mmol), RI (0.75 mmol), TMSN3(1.0 mmol), TBPB (1.0 mmol) in DME (2 mL) at rt for 5–20 min and then in toluene at 120 °C for 10 min under an N2atmosphere. Isolated yields 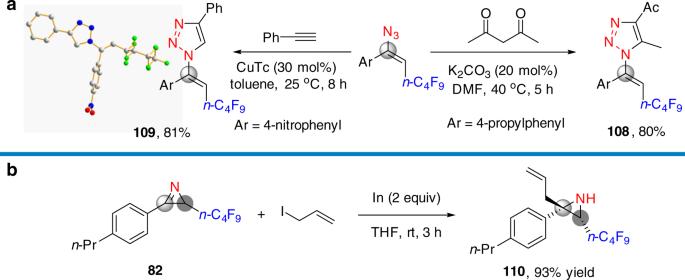Fig. 8 Further synthetic transformations.aSynthesis of 1,2,3-triazoles.bSynthesis of aziridine The solvent was then evaporated and the residue was purified by flash chromatography on silica gel using petroleum ether and EtOAc to give the corresponding product.